General heterostructure strategy of photothermal materials for scalable solar-heating hydrogen production without the consumption of artificial energy Solar-heating catalysis has the potential to realize zero artificial energy consumption, which is restricted by the low ambient solar heating temperatures of photothermal materials. Here, we propose the concept of using heterostructures of black photothermal materials (such as Bi 2 Te 3 ) and infrared insulating materials (Cu) to elevate solar heating temperatures. Consequently, the heterostructure of Bi 2 Te 3 and Cu (Bi 2 Te 3 /Cu) increases the 1 sun-heating temperature of Bi 2 Te 3 from 93 °C to 317 °C by achieving the synergy of 89% solar absorption and 5% infrared radiation. This strategy is applicable for various black photothermal materials to raise the 1 sun-heating temperatures of Ti 2 O 3 , Cu 2 Se, and Cu 2 S to 295 °C, 271 °C, and 248 °C, respectively. The Bi 2 Te 3 /Cu-based device is able to heat CuO x /ZnO/Al 2 O 3 nanosheets to 305 °C under 1 sun irradiation, and this system shows a 1 sun-driven hydrogen production rate of 310 mmol g −1 h −1 from methanol and water, at least 6 times greater than that of all solar-driven systems to date, with 30.1% solar-to-hydrogen efficiency and 20-day operating stability. Furthermore, this system is enlarged to 6 m 2 to generate 23.27 m 3 /day of hydrogen under outdoor sunlight irradiation in the spring, revealing its potential for industrial manufacture. Promoting industrial catalysis consumes a large amount of artificial energy, such as electricity [1] and fossil-derived energy [2] , which need artificial conversion and input for their final usage. Therefore, constructing artificial-energy-input-free catalysis is the key to human sustainable development. Sunlight-driven catalysis is a typical type of artificial-energy-input-free catalysis that has the potential to solve the energy bottleneck of catalysis [3] , [4] , [5] . At present, sunlight-driven catalysis mainly includes photocatalysis via sunlight-photogenerated carrier-chemical paths and photothermal catalysis via sunlight-hot carrier-chemical paths [6] , [7] , exhibiting great potential in many fields [8] , [9] . In addition to the above two kinds of sunlight-driven catalysis, using sunlight-converted thermal energy to drive thermal catalysis, that is, solar-heating catalysis, has aroused much attention [10] , [11] . In solar-heating catalysis, the photothermal material is the key for diverse solar-heating applications [12] , and it is challenged by achieving a high solar-heating temperature upon irradiation by diluted ambient sunlight [13] , [14] , [15] , [16] , [17] . In previous reports [18] , coordinated regulation of high solar absorption [19] and low thermal conductivity by materials such as black photothermal materials with porous [20] , amorphous [21] , and layered structures [22] was the main strategy used to improve solar-heating temperatures [23] , [24] . For example, a nanohybrid combining zeolitic imidazolate frameworks (ZIFs) and graphene was demonstrated to synergistically intensify sunlight absorbance (~98% solar-to-thermal conversion efficiency) and thermal energy insulation capability (ultralow thermal conductivity of ~0.2 W mK −1 ) to achieve a reported maximum solar-heating temperature of 120 °C under 1 sun illumination (equal to an energy density of 1 kW m −2 ) [25] , which is still too low to drive most thermocatalytic reactions. From the ideal artificial-energy-input-free catalysis design point of view, it is necessary to propose a concept to further improve the solar-heating temperatures. Hydrogen energy has been considered one of the foundations for future energy systems [26] , [27] , [28] . Owing to the storage limitations of hydrogen, such as high pressure, leakage, and extensive safety precautions, Olah proposed a methanol economy, as methanol can act as a hydrogen carrier in future hydrogen energy systems [29] , which has the merits of high hydrogen storage density (99 kg m −3 ), high degree of safety, low cost and compatibility with existing fossil energy systems [30] , [31] , [32] . However, hydrogen generation from methanol and water by methanol steam reforming (CH 3 OH + H 2 O → CO 2 + 3H 2 , MSR) requires a large-scale external energy input (16.47 kJ energy for 1 mol of H 2 ) [33] . A large amount of energy consumption has become the bottleneck for the large-scale application of methanol-hydrogen energy systems. Using sunlight to drive MSR is an attractive way to solve the artificial energy consumption problem [34] , [35] , [36] . As far as we know, the state-of-the-art sunlight-driven hydrogen production rate from methanol and water is ~46 mmol g −1 h −1 [37] , [38] , [39] , [40] , [41] , far behind industry requirements [42] , [43] . Therefore, development of an artificial-energy-input-free MSR mode with a greatly improved reaction rate is urgent for its applicability. Herein, taking a typical narrow-band gap photothermal material, Bi 2 Te 3 , as an example, we demonstrate a concept to increase the sunlight irradiation temperature of photothermal materials in which a heterogeneous Bi 2 Te 3 thin-film structure is synthesized on a Cu support (Bi 2 Te 3 /Cu) to simultaneously balance sunlight absorption and thermal radiation [22] , [44] . Sunlight absorption and thermal dissipation can be controlled by tuning the thickness of the Bi 2 Te 3 thin film, resulting in a 1 sun heating temperature of 317 °C, which is much higher than that of pure Bi 2 Te 3 (93 °C). Moreover, this strategy can also generally raise the 1 sun-heating temperatures of other photothermal materials to above 250 °C, and a reaction device based on Bi 2 Te 3 /Cu can heat catalysts to 305 °C under 1 sun irradiation. Furthermore, a soft templating method is developed to synthesize CuZnAl nanosheets, which have excellent thermocatalytic MSR activity and stability due to their ultrathin thickness, large specific surface area, and uniform elemental distribution. Consequently, without consuming artificial energy, CuZnAl nanosheets combined with the Bi 2 Te 3 /Cu-based device exhibit a solar-heating MSR performance that is far beyond all of sunlight-driven methanol-based hydrogen production systems reported to date. Moreover, a scalable model is constructed in this work, and it successfully produces 23.27 m 3 /day of hydrogen from MSR under 6 m 2 of outdoor sunlight irradiation in the spring. Using Bi 2 Te 3 /Cu to achieve a high solar-heating temperature Bi 2 Te 3 is a typical photothermal material with a narrow band gap (<0.2 eV) [45] , [46] that can nearly fully absorb the solar spectrum (Supplementary Fig. 1a, b ) and has a high carrier concentration of 0.84–1.11 × 10 19 cm −3 (Supplementary Fig. 1c ). Therefore, absorbed sunlight can be fully thermalized by this type of narrow-bandgap semiconductor via electron–phonon and electron–electron scattering [47] . For instance, Cheng et al. reported that Bi 2 Te 3 could convert up to 99% of solar energy into heat energy [48] . To achieve a high solar irradiation temperature, besides the superior solar-to-thermal conversion, it is also necessary to localize the sunlight-converted heat energy in Bi 2 Te 3 to reduce the amount of heat dissipation. Although vacuum protection was applied to cut off the heat conduction loss of the pure Bi 2 Te 3 film, the 1-sun (1 kW m −2 ) illumination temperature of the pure Bi 2 Te 3 film was only 93 °C (Supplementary Fig. 1d ). As a blackbody material (Fig. 1a ) [49] , the heat dissipation of the pure Bi 2 Te 3 film includes not only the heat conduction loss but also, importantly, the violent heat radiation loss caused by infrared light (IR) radiation (IR emissivity of 0.91, as shown in the Supplementary Information ) [50] . Therefore, minimizing the IR radiation of Bi 2 Te 3 is the key to increasing its solar irradiation temperature. The IR light irradiated by Bi 2 Te 3 is produced by lattice vibrations, and the lattice vibrations are proportional to the number of atoms in Bi 2 Te 3 [51] . From the physical principle, reducing the number of atoms in the Bi 2 Te 3 structure can weaken IR radiation, so our strategy involves synthesizing a Bi 2 Te 3 thin film to minimize the number of atoms and minimize the IR radiation, as shown in Fig. 1b . To achieve a low-IR radiation of the Bi 2 Te 3 thin-film structure, the supports used to deposit the Bi 2 Te 3 thin film also need to exhibit the low-IR radiation property. However, the supports used to deposit Bi 2 Te 3 thin films are usually silicon wafer, which is also a typical blackbody material with strong IR radiation capability and cannot be used as a support for reducing the IR radiation of the whole Bi 2 Te 3 thin-film structure [49] . Unlike blackbody materials, the highly conductive metal Cu contains a large number of nearly free electrons that can prevent the spillover of IR light [52] , making Cu have near-zero IR radiation (~3% IR emissivity, Supplementary Fig. 2 ) [53] , [54] . Therefore, Cu film is selected as the support to synthesize Bi 2 Te 3 thin films to make the hybrid have merits such as superior solar-to-thermal conversion from Bi 2 Te 3 and low-IR radiation from Cu [55] . By controlling the deposition time, the thickness of the Bi 2 Te 3 film on the Cu support was tuned to 3 μm (Fig. 1c ), 100 nm (Fig. 1d ), and 15 nm (Fig. 1e ). The interface structure is shown in Supplementary Fig. 3 . When the thickness of the Bi 2 Te 3 film in Bi 2 Te 3 /Cu was 3 μm, the 1-sun irradiation temperature was 97 °C with vacuum protection (Fig. 1f ), ~4 °C higher than that of pure Bi 2 Te 3 (93 °C, Supplementary Fig. 1d ) under the same conditions. Surprisingly, as the thickness of the Bi 2 Te 3 film in Bi 2 Te 3 /Cu was reduced to 100 nm, the 1-sun irradiation temperature of vacuum-protected Bi 2 Te 3 /Cu increased sharply to 317 °C (Fig. 1g ), which was not only 224 °C higher than that of pure Bi 2 Te 3 but also 197 °C higher than the reported highest 1-sun irradiation temperature of photothermal materials (120 °C), as far as we know [25] . This indicates that this strategy is useful for improving the solar-heating temperature of photothermal materials. Furthermore, when we reduced the thickness of Bi 2 Te 3 in Bi 2 Te 3 /Cu to 15 nm (Fig. 1e ), the 1-sun irradiation temperature was only 172 °C (Fig. 1h ), 145 °C lower than that of Bi 2 Te 3 /Cu with a Bi 2 Te 3 thickness of 100 nm. Therefore, the thickness of Bi 2 Te 3 has an important influence on the sunlight irradiation temperature of Bi 2 Te 3 /Cu. Fig. 1: Heterostructure strategy used to increase the solar irradiation temperature of Bi 2 Te 3 . a Map of the heat dissipation of the pure Bi 2 Te 3 film. b Synthesis of the Bi 2 Te 3 thin film on a Cu support (Bi 2 Te 3 /Cu). c – e SEM and TEM images of Bi 2 Te 3 /Cu with 3 μm-, 100 nm-, and 15 nm-thick Bi 2 Te 3 . f – h IR images of vacuum-protected Bi 2 Te 3 /Cu with 3 μm-, 100 nm-, and 15 nm-thick Bi 2 Te 3 . A CaF 2 glass fully covered each sample, and the vacuum degree of this equipment was 1.0 × 10 −3 Pa. The scale bars in c , d , and e are 1500, 30, and 5 nm, respectively. Full size image Thickness effect of Bi 2 Te 3 and the device based on Bi 2 Te 3 /Cu To explain the effect of Bi 2 Te 3 thin-film thickness on the sunlight irradiation temperature of Bi 2 Te 3 /Cu, we measured the light absorbed by the three Bi 2 Te 3 /Cu samples. For the 3 μm-, 100 nm-, and 15 nm-thick Bi 2 Te 3 thin films in Bi 2 Te 3 /Cu, Fig. 2a–c show absorbances in the sunlight region (400–2000 nm) of ~94%, 89%, and 43%, respectively. Bi 2 Te 3 has a narrow bandgap of <0.2 eV [45] , [46] ; thus, sunlight has enough energy to excite electron transitions in Bi 2 Te 3 [56] , [57] . And, the film thickness of Bi 2 Te 3 must be ≥100 nm to ensure more than 89% solar spectrum absorption. However, the absorption in the IR region was 4 and 5% when the thickness of the Bi 2 Te 3 thin film in Bi 2 Te 3 /Cu was 15 and 100 nm, respectively (Fig. 2b, c ), and it increased to 60% when the thickness of the Bi 2 Te 3 thin film was further increased to 3 μm (Fig. 2a ). As the absorptivity of light is equal to the emissivity of the corresponding light [54] , the 60% IR absorption showed that the IR emissivity of Bi 2 Te 3 /Cu with a 3 μm-thick Bi 2 Te 3 thin film is 60%, at least 10 times higher than that of Bi 2 Te 3 /Cu with 100 nm (5%)- and 15 nm (4%)-thick Bi 2 Te 3 thin films. For a more intuitive embodiment, we directly tested the IR radiation intensity (4–20 μm) of these samples heated to 93 °C. As shown in Fig. 2d, e, f , the IR radiation intensities in the range of 4 μm–20 μm are 248 W m −2 , 20.7 W m −2 , 16.6 W m −2 for Bi 2 Te 3 /Cu with 3 μm-, 100 nm-, and 15 nm-thick Bi 2 Te 3 thin films, respectively, significantly lower than the corresponding IR radiation of the pure Bi 2 Te 3 film of 377 W m −2 (Supplementary Fig. 1e ). 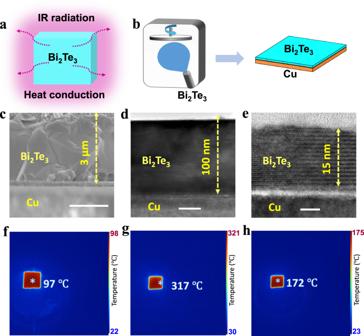Fig. 1: Heterostructure strategy used to increase the solar irradiation temperature of Bi2Te3. aMap of the heat dissipation of the pure Bi2Te3film.bSynthesis of the Bi2Te3thin film on a Cu support (Bi2Te3/Cu).c–eSEM and TEM images of Bi2Te3/Cu with 3 μm-, 100 nm-, and 15 nm-thick Bi2Te3.f–hIR images of vacuum-protected Bi2Te3/Cu with 3 μm-, 100 nm-, and 15 nm-thick Bi2Te3. A CaF2glass fully covered each sample, and the vacuum degree of this equipment was 1.0 × 10−3Pa. The scale bars inc,d, andeare 1500, 30, and 5 nm, respectively. Summarizing the solar absorptivity and IR emissivity listed in Supplementary Table 1 , the 100 nm-thick Bi 2 Te 3 layer can synergistically absorb 89% of sunlight and emit 5% of IR radiation; in other words, this 100 nm-thick Bi 2 Te 3 layer can absorb sunlight energy to the maximum extent and dissipate heat energy to the minimum extent so that the heat energy converted from sunlight is localized in the interior of the Bi 2 Te 3 layer, resulting in a high sunlight irradiation temperature. This method is also suitable for other narrow-band gap semiconductors, such as Ti 2 O 3 [58] , Cu 2 Se [59] , and Cu 2 S [60] . When we synthesized ~200 nm-thick Ti 2 O 3 , Cu 2 Se, and Cu 2 S on a Cu support (Supplementary Fig. 4 ), the Ti 2 O 3 /Cu, Cu 2 Se/Cu, Cu 2 S/Cu heterostructures showed 1-sun irradiation temperatures of 295, 271, and 248 °C (Fig. 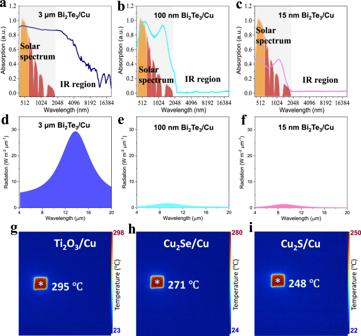Fig. 2: Thickness effect and universality of the heterostructure strategy. a–cNormalized light absorption spectra of Bi2Te3/Cu with 3 μm-, 100 nm-, and 15 nm-thick Bi2Te3layers.d–fIR radiation ranging from 4 μm to 20 μm for Bi2Te3/Cu with 3 μm-, 100 nm-, and 15 nm-thick Bi2Te3layers at 93 °C.g–iIR images of vacuum-protected Ti2O3/Cu, Cu2Se/Cu, Cu2S/Cu heterostructures. A CaF2glass fully covered each sample, and the vacuum degree of this equipment was 1.0 × 10−3Pa. 2g–i ), respectively, obviously higher than the 1-sun heating temperatures of pure Ti 2 O 3 (82 °C), Cu 2 Se (79 °C), and Cu 2 S (75 °C), as shown in Supplementary Fig. 5 . Meanwhile, different thicknesses of Ti 2 O 3 , Cu 2 Se, and Cu 2 S on the Cu support were synthesized (Supplementary Fig. 6 ), and the corresponding IR images (Supplementary Fig. 7 ) showed that the temperatures of those samples were all higher than the 1-sun heating temperatures of pure Ti 2 O 3 (82 °C), Cu 2 Se (79 °C), and Cu 2 S (75 °C), as shown in Supplementary Fig. 5 . These results confirm that the proper thickness is significant for narrow-bandgap semiconductors to have weak IR radiation while maintaining enough solar spectral absorption to achieve a high temperature in the device. Fig. 2: Thickness effect and universality of the heterostructure strategy. a – c Normalized light absorption spectra of Bi 2 Te 3 /Cu with 3 μm-, 100 nm-, and 15 nm-thick Bi 2 Te 3 layers. d – f IR radiation ranging from 4 μm to 20 μm for Bi 2 Te 3 /Cu with 3 μm-, 100 nm-, and 15 nm-thick Bi 2 Te 3 layers at 93 °C. g – i IR images of vacuum-protected Ti 2 O 3 /Cu, Cu 2 Se/Cu, Cu 2 S/Cu heterostructures. A CaF 2 glass fully covered each sample, and the vacuum degree of this equipment was 1.0 × 10 −3 Pa. Full size image As shown in Fig. 3a , hybridization of the Cu layer, Bi 2 Te 3 layer, vacuum layer, and glass layer was successively achieved on the outer surface of the reaction tube to form a device (named the Bi 2 Te 3 /Cu-based device). An optical image of a reaction tube is shown in Fig. 3b (Supplementary Fig. 8 ). Under 1-sun irradiation, the IR image shows that the inner temperature of the Bi 2 Te 3 /Cu-based device was as high as 307 °C (Fig. 3c ). As we loaded the CuZnAl catalyst in the Bi 2 Te 3 /Cu-based device, Fig. 3d shows that the temperature of the CuZnAl catalyst was higher than 200 °C at 0.5-sun irradiation, and the temperature reached 305 °C under 1-sun irradiation. The temperature of the CuZnAl catalyst-loaded Bi 2 Te 3 /Cu-based device was 230 °C higher than that of the CuZnAl catalyst directly irradiated by 1 sun (Supplementary Fig. 9 ). Fig. 3: Bi 2 Te 3 /Cu-based device. a Map of the Bi 2 Te 3 /Cu-based device loaded with catalysts for solar-heating MSR. b Photograph of the homemade Bi 2 Te 3 /Cu-based device. c Cross-sectional IR image of the Bi 2 Te 3 /Cu-based device under 1-sun irradiation. d Temperature of the CuZnAl catalyst loaded in the Bi 2 Te 3 /Cu-based device under different intensities of solar irradiation. Full size image Synthesis and characterization of the MSR catalyst: CuZnAl nanosheets With the device that can generate a high solar-heating temperature, we added commercial CuZnAl (C-CuZnAl, Supplementary Fig. 10 ) to the Bi 2 Te 3 /Cu-based device to test the sunlight-driven MSR performance. As shown in Supplementary Fig. 11 , the 1 sun-driven MSR H 2 generation rate achieved with C-CuZnAl was 79.3 mmol g −1 h −1 , which is much higher than the reported record photocatalytic MSR value (46.6 mmol g −1 h −1 ) [39] , thus highlighting the importance of the Bi 2 Te 3 /Cu-based device. To achieve better sunlight-driven MSR performance, more efficient catalysts for MSR need to be developed. In this work, polyvinylpyrrolidone (PVP, K30) was selected as a surfactant to synthesize this type of CuZnAl catalyst [61] . PVP was mixed with the CuZnAl precursor as a homogeneous solution, and then, the Na 2 CO 3 solution was dropped to precipitate CuZnAl oxides (Fig. 4a ). In the precipitation process, PVP was able to guide anisotropic growth and prevent aggregation. Consequently, we successfully controlled the morphology of CuZnAl oxides by tuning the PVP amount (Supplementary Fig. 12 , the optimized mass ratio of the PVP/CuZnAl precursor was 8). Supplementary Figure 13 shows that our synthesized sample could fully fill a 40 L bottle, revealing its scalable preparation. TEM imaging exhibits the porous nanosheet morphology of this sample (Fig. 4b ), so we labeled the sample CuZnAl NS. The elemental mapping images in Fig. 4c reveal that Cu, Zn, and Al are homogeneously dispersed in the CuZnAl NS. Nanoparticles with diameters of <5 nm were observed in the HRTEM image, with distinguishable lattice fringes assigned to Cu and ZnO (Fig. 4d ). The small sizes of Cu and ZnO provided more interfaces, so they were generally recognized as highly active sites for MSR [62] . The thickness of the CuZnAl NS was measured to be 3.2 nm (Fig. 4e ). According to the nitrogen adsorption–desorption measurements (Fig. 4f ), the CuZnAl NS exhibited a large specific surface area of 195.2 m 2 g −1 , four times larger than that of commercial C-CuZnAl (Supplementary Fig. 10 ), ensuring a large number of active sites for catalytic reactions. As a result, the hydrogen production rate of CuZnAl NS was 1.02 mol g −1 h −1 at 260 °C, quintupling the 0.2 mol g −1 h −1 hydrogen production rate of C-CuZnAl at 260 °C (Fig. 4g ), and the methanol conversion rate was 5.28% (Supplementary Fig. 14 ). Additionally, we tested CuZnAl NS for 20 days, and the hydrogen production rate at 260 °C was maintained at ~1 mol g −1 h −1 (Supplementary Fig. 15 ), indicating the excellent stability of CuZnAl NS. Fig. 4: Preparation and characterization of CuZnAl NS. a Schematic of the synthesis process for CuZnAl NS. TEM image b , elemental mapping image c , HRTEM image d , AFM image e , and nitrogen adsorption and desorption isotherm f of CuZnAl NS. 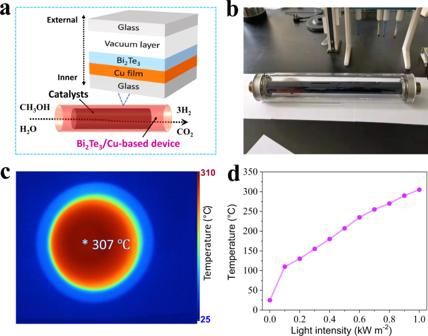Fig. 3: Bi2Te3/Cu-based device. aMap of the Bi2Te3/Cu-based device loaded with catalysts for solar-heating MSR.bPhotograph of the homemade Bi2Te3/Cu-based device.cCross-sectional IR image of the Bi2Te3/Cu-based device under 1-sun irradiation.dTemperature of the CuZnAl catalyst loaded in the Bi2Te3/Cu-based device under different intensities of solar irradiation. g Hydrogen production rate from the MSR of CuZnAl NS and C-CuZnAl at different temperatures. Test conditions: 10 mg of catalyst, 50 sccm of Ar, and 0.1 sccm of methanol (the volume ratio of methanol to water = 1:1.3). The scale bars in b , c , and d are 200, 500, and 2 nm, respectively. CuZnAl NS and C-CuZnAl are abbreviations for CuZnAl nanosheets and commercial CuZnAl, respectively. Full size image Solar-heating MSR Ten grams of CuZnAl NS was placed in the Bi 2 Te 3 /Cu-based device, and 0.0471 m 2 of sunlight irradiation was the only energy source. When the sunlight density was higher than 0.5 sun, a clear hydrogen signal appeared for the CuZnAl NS loaded in the Bi 2 Te 3 /Cu-based device, and the hydrogen generation rate increased to 3.1 mol h −1 (Fig. 5a ) under 1 sun irradiation, corresponding to 310 mmol g −1 h −1 and a methanol conversion rate of 45.34% (Supplementary Fig. 16 ). Meanwhile, the temperature of the CuZnAl NS loaded in the Bi 2 Te 3 /Cu-based device during solar-heating MSR is shown in Supplementary Fig. 17 . Comparatively, MSR showed a hydrogen production rate of zero, as the CuZnAl NS were directly irradiated by 1-sun irradiation without the device (Fig. 5a ). Since sunlight is the only energy source of the MSR catalytic reaction in solar-heating catalysis, as in the photocatalysis reaction, we listed the state-of-the-art sunlight-driven hydrogen production rates in Fig. 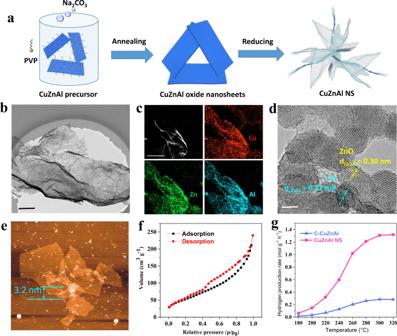Fig. 4: Preparation and characterization of CuZnAl NS. aSchematic of the synthesis process for CuZnAl NS. TEM imageb, elemental mapping imagec, HRTEM imaged, AFM imagee, and nitrogen adsorption and desorption isothermfof CuZnAl NS.gHydrogen production rate from the MSR of CuZnAl NS and C-CuZnAl at different temperatures. Test conditions: 10 mg of catalyst, 50 sccm of Ar, and 0.1 sccm of methanol (the volume ratio of methanol to water = 1:1.3). The scale bars inb,c, anddare 200, 500, and 2 nm, respectively. CuZnAl NS and C-CuZnAl are abbreviations for CuZnAl nanosheets and commercial CuZnAl, respectively. 5b and Table 1 for comparison with our data. 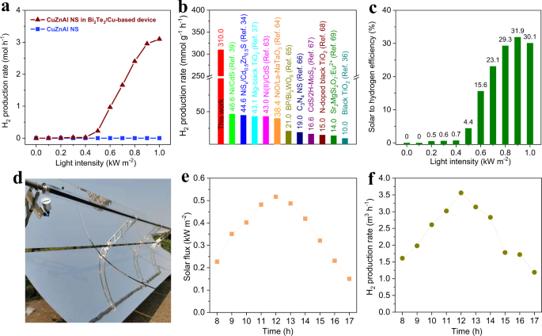Fig. 5: Solar-heating MSR performance of CuZnAl NS with a Bi2Te3/Cu-based device. aHydrogen production rates from the MSR of CuZnAl NS loaded in the Bi2Te3/Cu-based device and the device without CuZnAl NS under different sunlight irradiation.bVisual contrast diagram of the hydrogen production rates achieved under 1 sun illumination by the Bi2Te3/Cu-based device loaded with CuZnAl NS and those of other photocatalysts.cSTH efficiency of MSR achieved by the Bi2Te3/Cu-based device loaded with CuZnAl NS under different intensities of solar irradiation.dOptical image of the solar-heating system used for hydrogen production from MSR under ambient sunlight irradiation.eSolar flux on April 08, 2021, in Baoding City, China.fMSR hydrogen production rate as a function of time under ambient sunlight irradiation. CuZnAl NS is the abbreviation for CuZnAl nanosheets. Figure 5b and Table 1 confirm that our tested activity was at least 6 times the activity of the best sunlight-driven hydrogen production systems in the reported literature, e.g., Ni/CdS (46.6 mmol g −1 h −1 ) [39] , NiS x /Cd 0.5 Zn 0.5 S (44.6 mmol g −1 h −1 ) [34] , Mg-black TiO 2 (43.1 mmol g −1 h −1 ) [37] , Ni(II)/CdS (43 mmol g −1 h −1 ) [63] , NiO/LaNaTaO 3 (38.4 mmol g −1 h −1 ) [64] , BP/Bi 2 WO 6 (21.0 mmol g −1 h −1 ) [65] , C 3 N 4 (19 mmol g −1 h −1 ) [66] , CdS/2H-MoS 2 (16.6  mmol g −1 h −1 ) [67] , N-doped black TiO 2 (15 mmol g −1 h −1 ) [68] , Sr2MgSi2O7:Eu 2+ (14 mmol g −1 h −1 ) [69] , and black TiO 2 (10 mmol g −1 h −1 ) [36] . Based on the experimental data, the solar-to-hydrogen (STH) conversion efficiencies of CuZnAl NS in the Bi 2 Te 3 /Cu-based device were calculated to be 31.9% and 30.1% under 0.9- and 1-sun irradiation, respectively (Fig. 5c ). Note that the STH of our solar heating MSR is beyond the theoretical STH limit of photocatalytic MSR achieved through the route of photon-photogenerated electrons and holes-chemicals [70] . Ishii et al. reported that the average energy of photons in the solar spectrum is ~1 eV [71] . However, the reaction enthalpy of MSR is 0.086 eV per H (1/3 CH 3 OH (l) + 1/3 H 2 O (l)→ H 2 (g) + 1/3 CO 2 (g); detailed calculation shown in the Methods). Therefore, the STH ceiling of photocatalytic MSR under 1-sun illumination is 8.6% (0.086 eV/1 eV), equivalent to ~1/3 of the STH of our solar heating MSR system (30.1%) under 1-sun irradiation. This work reveals that solar heating catalysis via a solar-thermal energy-chemical route has an incomparable advantage over photocatalysis in reactions with a low energy barrier. Therefore, the Bi 2 Te 3 /Cu-based device with CuZnAl NS opens a pathway for efficiently achieving solar-driven hydrogen generation from methanol and water, in which solar heating is the only energy source used and has no energy supply from artificial input is needed, meaning that artificial energy is not consumed. In addition to the high hydrogen production rate, the ratio of CO 2 to CO 2 + CO in our solar-heating MSR strategy was higher than 99.2% under sunlight irradiation (Supplementary Fig. 18 ), indicating a low CO concentration in the hydrogen-producing process. Fig. 5: Solar-heating MSR performance of CuZnAl NS with a Bi 2 Te 3 /Cu-based device. a Hydrogen production rates from the MSR of CuZnAl NS loaded in the Bi 2 Te 3 /Cu-based device and the device without CuZnAl NS under different sunlight irradiation. b Visual contrast diagram of the hydrogen production rates achieved under 1 sun illumination by the Bi 2 Te 3 /Cu-based device loaded with CuZnAl NS and those of other photocatalysts. c STH efficiency of MSR achieved by the Bi 2 Te 3 /Cu-based device loaded with CuZnAl NS under different intensities of solar irradiation. d Optical image of the solar-heating system used for hydrogen production from MSR under ambient sunlight irradiation. e Solar flux on April 08, 2021, in Baoding City, China. f MSR hydrogen production rate as a function of time under ambient sunlight irradiation. CuZnAl NS is the abbreviation for CuZnAl nanosheets. Full size image Table 1 Sunlight-driven hydrogen generation from the MSR of CuZnAl NS loaded in a Bi 2 Te 3 /Cu-based device in comparison with the reported advanced sunlight-driven hydrogen generation systems. Full size table To test the capability of the Bi 2 Te 3 /Cu-based device for large-scale production (Supplementary Fig. 19 ), we prepared a scalable system, as shown in Fig. 5d . Its outdoor test was performed on 8 April 2021, with an ambient temperature of 6–21 °C and a sunlight intensity of 0.15–0.52 kW m −2 (Fig. 5e ) in the daytime in Baoding City of Hebei Province, China. To make the system work well in the morning and evening, the system was equipped with a parabolic reflector with a 6 m 2 irradiation area to concentrate sunlight to moderate its solar-heating MSR ability (Supplementary Movie 1 ). As shown in Fig. 5f , MSR took place at 8:00 A.M. with a hydrogen production rate of 1.61 m 3 h −1 . After that, the rate rose sharply, and the hydrogen production rate reached a peak of 3.56 m 3 h −1 at 12:00 P.M. and then gradually decreased to 1.19 m 3 h −1 at 17:00 P.M. The total amount of hydrogen produced daily was up to 23.27 m 3 under ambient sunlight irradiation, showing the potential of industrialization. In this work, we propose a solar-heating catalysis mode as a distinctive type of artificial-energy-input-free catalytic system. A heterostructure consisting of black photothermal materials, used to fully absorb sunlight, and a Cu support, used to weaken IR radiation, was used to increase the solar-heating temperature of photothermal materials. Taking Bi 2 Te 3 as an example, we found that the solar-spectrum absorption and IR radiation of the Bi 2 Te 3 film depended on the thickness of the Bi 2 Te 3 film. Consequently, hybridization of the 100 nm-thick Bi 2 Te 3 film with a Cu support showed a 1 sun-heating temperature of 317 °C with vacuum protection, 224 °C higher than that of pure Bi 2 Te 3 under the same conditions. This strategy is widely used in narrow-band gap materials, and the hybrids of Ti 2 O 3 /Cu, Cu 2 Se/Cu, and Cu 2 S/Cu exhibited 1 sun-heating temperatures of 295, 271, and 248 °C, respectively. A PVP-capped coprecipitation method was modified and used to synthesize CuZnAl nanosheets (CuZnAl NS) on a large scale with a thickness of 3.2 nm, a larger specific surface area of 195.2 m 2 g −1 , and a 5-nm Cu nanoparticle as benchmark catalysts for MSR. Finally, based on Bi 2 Te 3 /Cu, we synthesized a reaction device in which CuZnAl NS were heated to 305 °C under 1-sun irradiation, and 0.15 m 2 of 1 sun-heated MSR showed a hydrogen production rate of 3.1 mol h −1 , at least 6 times higher than that reported for sunlight-driven hydrogen production systems, with an STH efficiency of 30.1% and 20-day stability. Moreover, an industrial demo of our system driven by 6 m 2 of outdoor sunlight was able to generate 23.27 m 3 /day of H 2 from MSR. In these systems, the energy source used is only solar heating, and no other artificial energy is consumed. Deposition of the Bi 2 Te 3 film and synthesis of devices SP-0707AS magnetron sputtering was used to deposit the Bi 2 Te 3 film at a vacuum pressure lower than 7.0 × 10 −3 Pa, and a 4-axis rotation system was used to rotate the bases. Bi 2 Te 3 and Cu were used as targets; the working gas was Ar with 99.99% purity. The bases used in Figs. 1 – 3 and 5 were Cu films 20 × 20 × 0.1 mm in size, Cu films 20 × 20 × 0.1 mm in size, reaction tubes 250 mm in length and 30 mm in diameter, and stainless steel tubes 2000 mm in length and 42 mm in diameter, respectively. Before the deposition process, the bases were subsequently washed with deionized water, acetone, and ethanol. (1) For the deposition of the Bi 2 Te 3 film on the Cu film, glow discharge was applied to clean the Cu film, and then, the Bi 2 Te 3 film was deposited. Finally, the sample was removed after passive cooling. The power was 5 kW, the sputtering pressure was 9 × 10 −2 Pa, the bias voltage was 150 V, the sputtering temperature was 70 °C, and the sputtering times were 1 min and 6 min for Bi 2 Te 3 films with 15 nm and 100 nm thicknesses, respectively. For the 3 μm-thick Bi 2 Te 3 film, the sputtering pressure was 7 × 10 −1 Pa, and the sputtering time was 15 min. (2) For the synthesis of the Bi 2 Te 3 /Cu-based device involving the deposition of the Cu substrate and Bi 2 Te 3 film on the reaction tube, glow discharge was first applied to clean the glass tube. Then, the Cu layer was deposited by the Cu target and the Bi 2 Te 3 film was deposited by the Bi 2 Te 3 target in an orderly manner, with the sample being removed after passive cooling. The power was 5 kW, the sputtering pressure was 9 × 10 −2 Pa, the bias voltage was 150 V, the sputtering temperature was 70 °C, and the sputtering times for the Cu layer and Bi 2 Te 3 film were 12 min and 6 min, respectively. The thickness of the Cu layer was ~10 μm. The followed antireflection film and glass vacuum layer were provided by Hebei Scientist Research Experimental and Equipment Trade Co., Ltd. with a 1 × 10 −3 Pa pressure. The final product is shown in Fig. 3b . (3) For the synthesis of the device shown in Fig. 5d , involving the deposition of the Cu substrate and Bi 2 Te 3 film on a stainless steel tube, glow discharge was first performed to clean stainless steel tube, and then, the Cu layer was deposited by the Cu target and the Bi 2 Te 3 film was deposited by the Bi 2 Te 3 target in an orderly manner. Finally, the sample was removed after passive cooling. The power was 5 kW, the sputtering pressure was 9 × 10 −2 Pa, the bias voltage was 150 V, the sputtering temperature was 70 °C, and the sputtering times for the Cu layer and Bi 2 Te 3 film were 12 min and 6 min, respectively. The followed antireflection film and glass vacuum layer were provided by Hebei Scientist Research Experimental and Equipment Trade Co., Ltd. at a 1 × 10 −3 Pa pressure. The tubes were welded together to form a reaction tube 6 m in length for the outdoor test. Chemicals for catalysts Commercial copper nitrate (Cu(NO 3 ) 2 ), zinc nitrate hydrate (Zn(NO 3 ) 2 ·6H 2 O), aluminum nitrate hydrate (Al(NO 3 ) 3 ·9H 2 O), polyvinylpyrrolidone (PVP, K30), sodium borate, and sodium carbonate were purchased from Sinopharm Co., Ltd. The chemicals were all used without any further treatment. Catalyst preparation (CuZnAl NS, C-CuZnAl) A total of 375.7 g of Cu(NO 3 ) 2 , 297.4 g of Zn(NO 3 ) 2 ·6H 2 O, and 125.1 g of Al(NO 3 ) 3 ·9H 2 O were dissolved in 20 L of deionized water (containing 760 g of sodium borate). Then, 32 L of 150 mg mL −1 PVP aqueous solution was added to the above solution. The mixture solution was denoted solution A. Then, 0.2 M aqueous Na 2 CO 3 (10 L) was prepared and denoted solution B. Solution B was slowly added to solution A under stirring at 65 °C. The mixture solution was further stirred for 1 h and aged for 16 h at 65 °C. The precipitate was collected by centrifugation, washed with water three times, and dried by freeze-drying. Then, CuZnAl NS were obtained by calcination at 400 °C in air for 6 h and reduced in 10% H 2 /Ar at 300 °C for 10 h. C-CuZnAl was prepared by the coprecipitation method. Typically, 37.512 g of Cu(NO 3 ) 2 , 29.749 g of Zn(NO 3 ) 2 6H 2 O, and 12.504 g of Al(NO 3 ) 3 9H 2 O were dissolved in 200 mL of deionized water. After stirring for 1 h, the resulting solution and Na 2 CO 3 aqueous solution (0.2 M; 1 L) were added dropwise and stirred at 65 °C for 1 h. After holding at 65 °C for 4 h and ageing for 7 h, the resulting precipitate was washed several times with deionized water and then fast-frozen in liquid nitrogen. The frozen cube was freeze-dried at −55 °C and then calcinated in air at 400 °C for 6 h to obtain Cu-Zn-Al-based oxides. Finally, the products were reduced to 10% H 2 /Ar at 300 °C for 10 h and named C-CuZnAl. We tested the density of both CuZnAl NS and C-CuZnAl. The density of the CuZnAl NS powder was ~0.12 g cm −3 , and that of the C-CuZnAl powder was ~0.795 g cm −3 . STH calculation For the STH calculation, a Bi 2 Te 3 /Cu-based device with an irradiation area of 0.0471 m 2 was used in this experiment, and 10 g of CuZnAl NS fully filled the inner space of this device. In this test, methanol and water were mixed as a solution with a methanol to water volume ratio = 1:1.6, and the mixed solution was then pumped into the system. To analyse the hydrogen gas product, we first removed CO 2 from the produced gas through a NaOH solution (5 M), and a flowmeter (MV-192-H2, Bronkhorst) was used to measure the flow rate, which was recognized as the rate of hydrogen production. The STH efficiency of hydrogen generation from MSR was calculated as follows: 
    STH=(Δ H×ε /24.5)/(I× S× 3600)
 (1) The enthalpy change energies of methanol, CO 2 , H 2 , and H 2 O were −201.083, −393.505, 0, and −241.818 kJ mol −1 , respectively. ΔH is the reaction enthalpy change of methanol dehydrogenation (1/3 CH 3 OH (l) + 1/3 H 2 O (l)→ H 2 (g) + 1/3 CO 2 (g), ΔH = 16.47 KJ mol −1 ), ε (L) is the amount of H 2 generated per hour detected by a flowmeter (MV-192-H2), I is the light intensity (kW m −2 ), and S is the irradiated area of catalysts (0.0471 m −2 ). The calculation details and data are shown in Supplementary Fig. 20 . As 1 eV = 1.6 × 10 −19 J, the ΔH per H 2 was calculated to be 16.47 KJ/(1.6 × 10 −19 *6.02 × 10 23 ) = 0.171 eV; therefore, the Δ H per H was calculated to be 0.171 eV/2 = 0.086 eV.